Glycosphingolipid-functionalized nanoparticles recapitulate CD169-dependent HIV-1 uptake and trafficking in dendritic cells Ganglioside GM3, a host-derived glycosphingolipid incorporated in the membrane of human immunodeficiency virus-1 (HIV-1) viral particles, mediates interactions between HIV-1 and Siglec1/CD169, a protein expressed on dendritic cells (DCs). Such interactions, which seem to be independent of viral envelope glycoprotein gp120, are poorly understood. Here we develop a model system consisting of self-assembled artificial virus nanoparticles (AVNs) that are free of viral glycoproteins or other host-derived glycolipids and glycoproteins. These plasmonic AVNs contain a membrane of defined composition wrapped around a solid metal core. GM3-containing AVNs are captured by CD169-expressing HeLa cells or mature DCs, and are sequestered within non-lysosomal tetraspanin-positive compartments. This distribution is reminiscent of CD169-dependent HIV-1 sequestration in mature DCs. Our results highlight GM3–CD169 binding as a gp120-independent signal for sequestration and preservation of HIV-1 infectivity. They also indicate that plasmonic AVNs offer improved features over liposome-based systems and represent a versatile tool for probing specific virus–cell interactions. Virions are endogenous smart nanoparticles (NPs) that are evolutionarily optimized to achieve efficient reproduction in host cells. The viral surface plays a crucial role in establishing successful infection since it facilitates the binding of virus particles to the host cell and the subsequent initiation of an uptake programme that results in the delivery of the viral genetic content to the intracellular virus replication machinery [1] . Many of these interactions are facilitated by specific virus-encoded proteins, such as gp120 (human immunodeficiency virus-1 (HIV-1) envelope glycoprotein) in the case of productive (or cis) HIV-1 infection of CD4 + T cells and macrophages [2] , [3] , [4] . There is, however, a growing body of evidence that some infection mechanisms also depend critically on the composition of the viral lipidome [5] . In particular, host-derived glycosphingolipids incorporated in the virion play a central role for HIV-1 uptake and transmission by mature dendritic cells (DCs), a DC-mediated HIV-1 transinfection pathway [6] , [7] , [8] , [9] , [10] . The GSL that mediates the glycoprotein-independent interactions between HIV-1 and mature DCs was identified as monosialodihexosylganglioside (GM3) [8] , [11] , and the type 1 interferon-inducible Siglec1, CD169, has been identified as the corresponding receptor that recognizes GM3 present in the membrane of HIV-1 particles [9] , [12] . Furthermore, virus particles captured by CD169 in a GM3-dependent manner are sequestered in non-lysosomal compartments, and on initiation of DC–T cell contacts transferred to the DC–T cell synaptic junction, termed ‘virological synapse’ [13] . Since the cytoplasmic tail of CD169 lack any known endocytic motifs, many details of the mechanisms underlying CD169-mediated HIV-1 uptake and subsequent trafficking to DC–T cell virological synapses remain currently unclear. The latter is—at least in part—due to experimental complications associated with a systematic investigation of the role of individual host-encoded viral surface functionalities in transinfection. One particular challenge is that the compositional complexity of both cellular and viral surfaces gives rise to a multitude of potential interactions that can be both physical and chemical in nature and which are difficult to decouple in conventional virus models [14] . A second complication is that mechanistic information about the cellular machinery orchestrating the virus trafficking is best obtained by single virus trafficking [15] , [16] , [17] . This approach requires, however, bright labels that facilitate an optical tracking with high-temporal resolution, ideally without limitation in maximum observation time. Different virus model systems have been developed for delivery purposes [18] , [19] as well as for structural [20] or mechanistic studies [21] . Successful realizations include virus-like particles (VLPs) [22] , [23] , virus-based NPs [21] , [24] , liposomes [25] , [26] , [27] , and hybrid systems in which biomolecules are combined with inorganic NPs to reproduce viral functionality [19] , [24] , [28] , [29] . None of the systems implemented so far, however, fulfill all the specific requirements with regard to size, transducing capability, surface composition and engineerability to characterize the mechanistic role of GM3 in the membrane of the HIV-1 virion. For instance, HIV-1 Gag VLPs [30] , [31] , [32] , which are common tools for characterizing the role of non-virus-encoded host cell surface functionalities, are immature virion cores wrapped in a lipid bilayer derived on budding from a virus-producer cell and can contain host-derived membrane glycoproteins in addition to a broad range of different (glyco)lipids [33] . These additional groups can compete or interfere with the biological functionality of GM3. In this manuscript, we overcome this complication and characterize the specific functionality of GM3 as a potential viral surface ligand using an approach of reverse nanoengineering. We demonstrate with artificial virus NPs (AVNs), which contain a membrane of defined composition wrapped around a metal nanoparticle core, that the recognition of GM3 through cell surface CD169 is sufficient to facilitate a specific binding of AVNs and virus particles to host cells. Unlike GM3-containing liposomes, the GM3-functionalized AVNs induce a temporospatial distribution that is distinctly different from conventional NP endocytosis and that results in an enrichment of AVNs in peripheral, tetraspanin-positive, non-lysosomal compartments. Design and fabrication of artificial virus NPs HIV-1 particle assembly and budding can occur on expression of Gag alone in the absence of other viral proteins in host cells. The mature virus particle has a typical size between 120–150 nm [34] , [35] , contains ~\n2,500 Gag molecules and is wrapped in a lipid bilayer that the virus acquires from the plasma membrane during budding from the host cell (reviewed in ref. 36 ). The Gag polyprotein is proteolytically cleaved into six structural proteins, matrix (MA), nucleocapsid, capsid, p6 and two spacer proteins, SP1 and SP2 during the virus maturation step [37] . Schematic illustrations of the mature virus structure containing the MA protein-enclosed capsid shell with the nucleocapsid-coated viral RNA and the AVN models to mimic it are shown in Fig. 1a,b , respectively. Our AVN design is based on a self-assembled lipid layer around an 80 nm diameter noble metal NP that serves as an analogue of the lipid enclosed core formed by association of basic amino-acid residues in MA with the inner leaflet of the phosphatidylinositol 4,5-bisphosphate [PI(4,5)P 2 ]-enriched lipid bilayer [36] . The lipid layer emulates the virus membrane but is entirely free of proteins and can be engineered with a defined lipid composition, ligand density and controllable surface charge. In this work, we are particularly interested in GM3-containing AVNs for a selective investigation of GM3 interactions with CD169 under well-defined conditions in the absence of potential interferents. We chose gold (Au) as core material since it provides the assembled AVNs with mechanical stiffness [38] , [39] and, at the same time, allows high contrast optical imaging in optical, electron, and x-ray microscopy [40] , [41] . The optical response of spherical Au nanoparticles (Au NPs) is dominated by localized surface plasmon resonances in the visible range of the electromagnetic spectrum [42] . A resonant excitation of the LSPR in an 80 nm Au NP is associated with a scattering cross-sections of approximately σ ≈2.3 × 10 −10 cm −2 (ref. 43 ). This huge elastic scattering efficiency, which is orders of magnitude larger than conventional fluorescence cross-sections, facilitates single particle detection entirely free from blinking or bleaching in conventional darkfield microscopy [41] , [44] . Their unique photophysical stability together with their programmable surface properties make Au NPs the core of choice for AVNs in optical studies. 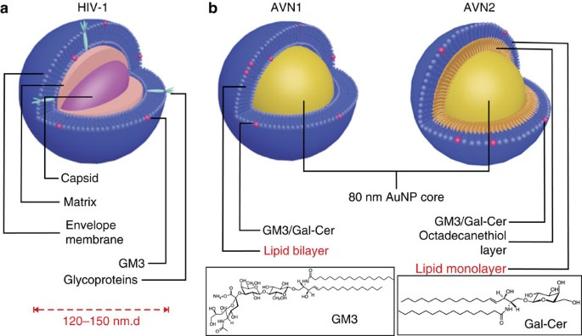Figure 1: Design of AVNs. (a) Scheme of HIV-1 structure. HIV-1 is composed of a host-derived lipid bilayer membrane wrapped around a protein MA core that contains the viral RNA. Major lipid components of the viral membrane are described inTable 1. The viral membrane contains additional lipids, including GM3, albeit with significantly lower concentration. Another membrane component is the virus-encoded glycoprotein gp120. (b) Scheme of minimalistic artificial model systems, AVN1 (left) and AVN2 (right). Both AVNs are assembled from 80 nm Au NP cores and comprise a self-assembled lipid membrane. AVN1 contains a lipid bilayer, whereas AVN2 contains a lipid monolayer anchored in a self-assembled octadecanethiol layer. The thiol covalently attaches to the NP surface. Figure 1: Design of AVNs. ( a ) Scheme of HIV-1 structure. HIV-1 is composed of a host-derived lipid bilayer membrane wrapped around a protein MA core that contains the viral RNA. Major lipid components of the viral membrane are described in Table 1 . The viral membrane contains additional lipids, including GM3, albeit with significantly lower concentration. Another membrane component is the virus-encoded glycoprotein gp120. ( b ) Scheme of minimalistic artificial model systems, AVN1 (left) and AVN2 (right). Both AVNs are assembled from 80 nm Au NP cores and comprise a self-assembled lipid membrane. AVN1 contains a lipid bilayer, whereas AVN2 contains a lipid monolayer anchored in a self-assembled octadecanethiol layer. The thiol covalently attaches to the NP surface. Full size image Different experimental strategies have been developed for creating lipid layers around NP cores with different sizes [23] , [45] , [46] , [47] , [48] , [49] . For the relatively large NPs of our AVN design, two strategies in particular are promising ( Fig. 2 ). Strategy 1 (S1) is based on a lipid encapsulation approach that traps Au NPs within unilamellar vesicles [46] . Strategy 2 (S2) incorporates the lipids with their hydrophobic tail into an octadecanethiol brush assembled on the surface of Au NPs [45] . While S1 leads to a complete bilayer membrane, S2 embeds a single layer of lipids into a self-assembled monolayer of octadecanethiols through their hydrophobic lipid tails. Both, S1 and S2, achieve a presentation of GM3 on the AVN surface with the sialic acid containing sugar head group pointing into the solution. In the following, we refer to the artificial virus NPs obtained through these two strategies as AVN1 and AVN2, respectively. Although S2 is synthetically simpler and more efficient than S1, lipid mobility and density obtained via S2 are anticipated to differ from those of the native bilayer membrane of enveloped virus particles. A priori it was, therefore, unclear if AVN2 could successfully mimic virus-like-behaviour and we consequently pursued and evaluated both strategies. 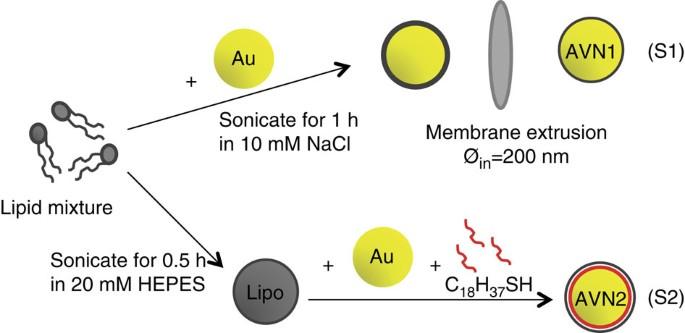Figure 2: Strategies for AVN fabrication. Schematic overview of fabrication strategies S1 (top) for AVN1 and S2 (bottom) for AVN2. The encapsulation strategy S1 traps Au NPs in liposomes formedin situ, whereas in S2 pre-formed liposomes act as lipid reservoir for the assembly of lipid membranes around octadecanethiol-coated Au NPs in a one-pot process. Lipo, Liposome. Figure 2: Strategies for AVN fabrication. Schematic overview of fabrication strategies S1 (top) for AVN1 and S2 (bottom) for AVN2. The encapsulation strategy S1 traps Au NPs in liposomes formed in situ , whereas in S2 pre-formed liposomes act as lipid reservoir for the assembly of lipid membranes around octadecanethiol-coated Au NPs in a one-pot process. Lipo, Liposome. Full size image HIV-1 preferentially buds from lipid rafts so that the host-derived viral membrane is enriched in lipids with saturated fatty acids, glycosphingolipids [50] , and cholesterol [51] . We simplified the membrane composition for the AVNs and used a limited number of lipids of comparable size that provide similar physicochemical properties as the virus membrane. The compositions of the viral membrane and of the AVN membranes used in this work are summarized in Table 1 . We chose dipalmitoylphosphatidylcholine containing two hydrophobic fatty acid chains and cholesterol as main components of the investigated membranes and integrated small quantities of phosphatidylserine to provide a negative surface charge comparable to that on HIV-1 particles [52] , [53] . In addition, TopFluor-labelled cholesterol molecules were incorporated into the membrane to monitor AVN formation via fluorescence microscopy. Either 3 mol% GM3 or α-Galactosylceramide (Gal-Cer) was added to test the role of these lipids for binding CD169. We included Gal-Cer as control in our studies since it is chemically similar to GM3 but does not contain any sialic acid residues and, thus, was shown previously to not bind CD169 (ref. 8 ). Table 1 Lipid membrane composition of HIV-1 and AVN particles in molar percentage. Full size table Characterization of AVNs We characterized the generated AVNs by measuring their hydrodynamic diameters and zeta potentials (ZP) ( Fig. 3a,b ). The hydrodynamic radius, reported as the peak in the size distribution obtained through dynamic light scattering, for GM3-containing AVN1 is r hyd (AVN1)=77.8±5.3 nm (s.d.) compared with r hyd (AVN2)=50.7±3.0 nm (s.d.) for GM3-containing AVN2. The observed difference in r hyd between AVN1 and AVN2 is too large to be accounted for only by differences in the membrane shell. Instead, the measured size difference indicates some self-association of the 80 nm Au NPs in the case of AVN1. Consistent with an increased level of NP clustering [41] , [54] , [55] , the ultraviolet–visible spectra (see Supplementary Fig. 1 ) confirm a red-shift of the ensemble-averaged plasmon resonance wavelength of ~\n8 nm for AVN1 when compared with AVN2. Both of the AVNs have zeta potentials between −20 and approximately −30 mV, which is close to the published value for HIV-1 particles of −20 mV under identical experimental conditions [52] . Due to their resonant interaction with the incident light, the Au NPs used in this work are extraordinarily bright and have a characteristic green–orange colour. Liposomes and other organic contaminations with comparable sizes, in contrast, are dim (see Supplementary Fig. 2 ) or appear as broadband scatterers, which makes them easily discernable from metal NPs. Correlated darkfield/fluorescence microscopy (see Supplementary Fig. 3 ) is, therefore, an appropriate method for validating successful lipid wrapping around the NPs. 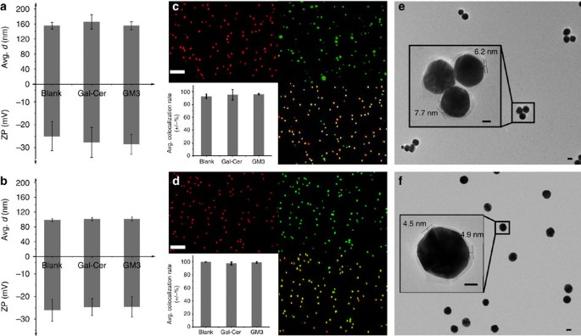Figure 3: Characterization of AVNs. ZP and average hydrodynamic diameter of (a) AVN1 and (b) AVN2 without glycosphingolipids (blank) or containing 3% Gal-Cer, or 3% GM3. The presented data were obtained from three independent experiments. Darkfield image, fluorescence image, overlay and colocalization statistics (clockwise top left to bottom right) for (c) AVN1 and (d) AVN2. A quantity of 1,000 particles were evaluated for each colocalization statistics. Representative TEM image of (e) AVN1 and (f) AVN2. The insets in (e) and (f) contain magnified views of selected AVNs, which show a distinct corona formed by the self-assembled lipids around the NPs. Scale bars, 10 μm in (c) and (d) and 20 nm in (e) and (f). Figure 3c,d show darkfield and fluorescence images of surface-immobilized AVN1 and AVN2 for representative preparations. Consistent with a successful formation of AVNs that contain both lipid and noble metal NP components, the images show >90% colocalization of fluorescence and darkfield signals for all AVN preparations. The exact colocalization statistics for ~\n1,000 particles of each type are summarized in the insets. Control experiments performed with pegylated Au NPs incubated with TopFluor cholesterol in the absence of lipids did not yield any measurable fluorescence signal (see Supplementary Fig. 4 ). High-resolution TEM images of AVN1 and AVN2 ( Fig. 3e,f ) show a distinct corona around the NPs, which is an additional proof of successful membrane assembly around the NPs. For AVN2, the corona is 4–5 nm thin. Together with the small difference between r hyd (AVN2) and the hydrodynamic radius of the citrate stabilized Au NPs ( r hyd =49.0±1.2 nm (s.d. )), the thin corona indicates the addition of a single-lipid layer to the octadecanethiol-functionalized NPs in the AVN2 assembly process. Figure 3: Characterization of AVNs. ZP and average hydrodynamic diameter of ( a ) AVN1 and ( b ) AVN2 without glycosphingolipids (blank) or containing 3% Gal-Cer, or 3% GM3. The presented data were obtained from three independent experiments. Darkfield image, fluorescence image, overlay and colocalization statistics (clockwise top left to bottom right) for ( c ) AVN1 and ( d ) AVN2. A quantity of 1,000 particles were evaluated for each colocalization statistics. Representative TEM image of ( e ) AVN1 and ( f ) AVN2. The insets in ( e ) and ( f ) contain magnified views of selected AVNs, which show a distinct corona formed by the self-assembled lipids around the NPs. Scale bars, 10 μm in ( c ) and ( d ) and 20 nm in ( e ) and ( f ). Full size image Consistent with the larger r hyd and relative spectral red-shift for AVN1 when compared with AVN2, the TEM images show mostly small clusters for AVN1, whereas for AVN2, individual Au NPs are predominantly observed. Although AVN1 preparations show some partial NP self-association, the average sizes of both AVN1 and AVN2 overlap with the natural size distribution of a HIV-1 virion. We conclude that based on the physical parameters of size, shape and surface charge, both S1 and S2 represent viable synthetic strategies for AVNs. We also tested the mechanical stiffness of individual VLPs and AVN2 particles through atomic force microscopy nanoindentation measurements and found that AVN particles are stiffer than VLPs or liposomes. These findings are consistent with previous nanoindentation studies that reported a Young’s modulus in the few GPa range and above [56] for biomolecule-loaded Au NPs and Young’s moduli of ~\n950 MPa or ~\n440 MPa for immature and mature HIV virions [39] , respectively. Liposomes are softer than both AVNs and virus particles; egg-PC cholesterol (1:1) liposomes, for instance, have a Young’s modulus of ~\n13 MPa [57] . GM3-mediated temporospatial distribution of VLPs VLPs are currently the model systems of choice for investigating the viral glycoprotein-independent capture of HIV-1 particles [7] , [8] , [9] , whose behaviour defines logical benchmarks for the evaluation of our reverse engineering strategy. In a first round of calibration experiments, we evaluated the binding specificity of VLPs in HeLa cells transduced to constitutively express CD169 (HeLa/CD169). Cells were incubated for 10 min with 1 × 10 10 ml −1 VLPs in Dulbecco’s modified Eagle medium (DMEM), washed and transferred to the fluorescence microscope for an optical inspection of the binding. We found that VLPs bound efficiently to HeLa/CD169 ( Fig. 4a ) but not to CD169-negative parental HeLa cells ( Fig. 4b ). This selective binding confirms that VLP binding is CD169 specific. Previous studies by Puryear et al . [13] and Izquierdo-Useros et al . [7] , [9] have demonstrated that GM3-mediated interactions of VLPs and infectious HIV-1 particles with CD169 on mature DCs induced a polarized virus distribution that resulted in an accumulation of the particles in non-lysosomal focal spots with preferential localization at the cell periphery. This characteristic spatial distribution was typically observed within 1–2 h after virus binding with the exact time depending on the particle concentration. Interestingly, we observed a similar clustering of VLPs in HeLa/CD169 only when the cells were cultured for additional time after exposure to the VLPs. While the VLPs are initially randomly distributed across the surface of HeLa/CD169 cells ( Fig. 4a ), they experience a spatial redistribution as a function of time. In ~\n1/3 of the cells, this redistribution culminates after 20 h in a strong local enrichment of VLPs in spatially confined spots. In good agreement with previous observations in DCs [7] , [9] , [13] , the locations of VLP enrichment do not co-stain with LysoTracker, which is a marker for acidified intracellular compartments, and the VLP enriched spots are often located at the cell periphery ( Fig. 4c,d ). We augmented the VLP tracking with simultaneous spatial mapping of the CD169–mCherry fusion protein and observed strong enrichment of CD169–mCherry at the site of VLP clustering ( Fig. 4e–g ), consistent with a role of CD169 as the receptor for HIV Gag VLPs. 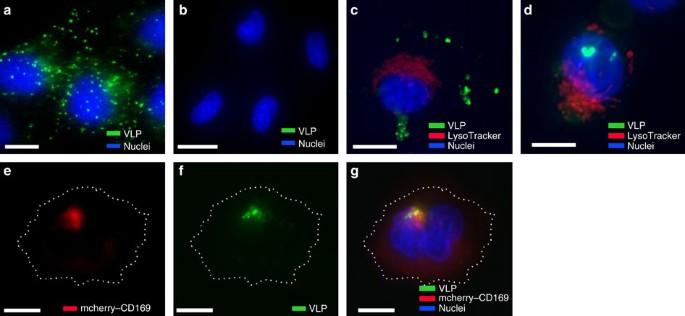Figure 4: Spatial redistribution of HIV Gag–eGFP VLPs after binding to HeLa/CD169 cells. The VLPs selectively bind to (a) HeLa/CD169 cells but not to (b) parental HeLa cells after 10 min of incubation. (c,d) Twenty hours after binding to HeLa/CD169, the initially randomly distributed VLPs are enriched in peripheral compartments that do not co-stain with lysosome tracker. Fluorescence images of (e) CD169–mCherry, (f) VLP and (g) overlay 20 h after initial incubation with HIV Gag–eGFP VLPs. The fluorescence data show a strong optical colocalization of CD169 and VLPs. The VLP segregation was confirmed in two independent imaging experiments. Scale bars, 5 μm. Figure 4: Spatial redistribution of HIV Gag–eGFP VLPs after binding to HeLa/CD169 cells. The VLPs selectively bind to ( a ) HeLa/CD169 cells but not to ( b ) parental HeLa cells after 10 min of incubation. ( c , d ) Twenty hours after binding to HeLa/CD169, the initially randomly distributed VLPs are enriched in peripheral compartments that do not co-stain with lysosome tracker. Fluorescence images of ( e ) CD169–mCherry, ( f ) VLP and ( g ) overlay 20 h after initial incubation with HIV Gag–eGFP VLPs. The fluorescence data show a strong optical colocalization of CD169 and VLPs. The VLP segregation was confirmed in two independent imaging experiments. Scale bars, 5 μm. Full size image CD169-mediated uptake and sequestration of GM3-AVNs In the next step, we verified whether GM3-containing AVNs reproduce the observed VLP behaviour. First, we tested if nanoconjugated GM3 is a ligand for CD169 by quantifying the binding efficacies of GM3 and Gal-Cer-containing AVNs and of blank controls. HeLa and HeLa/CD169 cells were incubated with 5 × 10 8 ml −1 AVNs in DMEM for 10 min, washed to remove unbound particles and inspected via darkfield microscopy. Interestingly, only GM3-containing AVN1 ( Fig. 5a ) and AVN2 ( Fig. 5b ) but not Gal-Cer-containing AVN1 ( Fig. 5c ) or AVN2 ( Fig. 5d ) bind to HeLa/CD169 cells. GSL-free blank AVN1 ( Fig. 5e ) or AVN2 ( Fig. 5f ) also did not bind to HeLa/CD169 cells. In additional control experiments, we verified that GM3-containing AVNs do not bind to HeLa cells (see Supplementary Fig. 5e ). Together, these observations confirm that GM3-functionalized AVNs bind specifically to CD169. 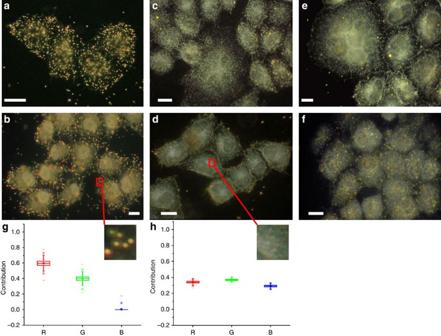Figure 5: Binding of AVNs to HeLa/CD169 cells is GM3 specific. (a) Darkfield image of HeLa/CD169 cells after 10 min of incubation with AVN1 particles containing 3% GM3. AVN1 binds efficiently to HeLa/CD169. (b) AVN2 particles containing 3% GM3 also show efficient binding to HeLa/CD169 under otherwise identical conditions. In contrast, (c) AVN1 or (d) AVN2 particles with 3% Gal-Cer show no binding to HeLa/CD169 cells. Similarly, the binding of (e) AVN1 blanks or (f) AVN2 blanks (no GM3 or Gal-Cer) to HeLa/CD169 is negligible. (g) Relative intensity distribution on the red (R), green (G) and blue (B) colour channels of a digital camera for an AVN-bound cell surface (see inset) and (h) for control cell surface void of AVNs. Scale bars, 10 μm. GM3 binding specificity studies were independently repeated >3 times. Figure 5: Binding of AVNs to HeLa/CD169 cells is GM3 specific. ( a ) Darkfield image of HeLa/CD169 cells after 10 min of incubation with AVN1 particles containing 3% GM3. AVN1 binds efficiently to HeLa/CD169. ( b ) AVN2 particles containing 3% GM3 also show efficient binding to HeLa/CD169 under otherwise identical conditions. In contrast, ( c ) AVN1 or ( d ) AVN2 particles with 3% Gal-Cer show no binding to HeLa/CD169 cells. Similarly, the binding of ( e ) AVN1 blanks or ( f ) AVN2 blanks (no GM3 or Gal-Cer) to HeLa/CD169 is negligible. ( g ) Relative intensity distribution on the red (R), green (G) and blue (B) colour channels of a digital camera for an AVN-bound cell surface (see inset) and ( h ) for control cell surface void of AVNs. Scale bars, 10 μm. GM3 binding specificity studies were independently repeated >3 times. Full size image We included a comparison of the spectral content of AVNs and cellular background by analysing the relative intensity distribution on the red (R), green (G) and blue (B) colour channels of the digital camera used to acquire the cell images. While the intensity of the cellular background is equally distributed across the R, G, B channels, the relative contributions from the R and G channels are locally increased in areas containing AVNs. We conclude that, due to their spectral characteristics and their high intensity (see insets), AVNs built around an 80 nm Au core can be differentiated with high fidelity even from grainy background in the investigated single-cell layer. We took advantage of the large optical cross-sections of GM3-functionalized AVNs to determine their spatial distribution in HeLa/CD169 cells 20 h after initial AVN binding. These experiments revealed a characteristic spatial redistribution of the AVNs from an initial random distribution to a preferential spatial enrichment in discrete spots at the cell periphery. The representative darkfield images of GM3-containing AVN1-treated ( Fig. 6a,b ) and AVN2-treated ( Fig. 6c,d ) HeLa/CD169 cells acquired 20 h after AVN exposure illustrate the formation of distinct NP clusters at the cell periphery. In the case of AVN2, we also performed fluorescence staining experiments to image the acidified membrane compartments and the cell nuclei ( Fig. 6e,f ). The correlated darkfield/fluorescence images reveal that the locations of high AVN concentration do not colocalize with LysoTracker. The preferential localization of AVN clusters at the HeLa/CD169 cell periphery in LysoTracker-negative compartments excludes conventional lysosomal compartments as origin of the large-scale AVN clustering, similar to the localization pattern observed with HIV Gag–eGFP VLPs. As in the case of the VLPs, we observed this phenotype in ~\n1/3 of all investigated cells. We attribute the variability in the cellular response to AVNs and VLPs to the intrinsic heterogeneity of immortalized cancer cell lines [58] , [59] , as well as to variations in the CD169 expression level on the single-cell level. The observation of similar spatiotemporal distributions for both AVN1 and AVN2 implies that the intact lipid bilayer membrane of AVN1 is not required to trigger GM3–CD169-mediated cellular processes, but that the presentation of GM3 in a single leaflet tethered to a solid core, as is the case for AVN2, is sufficient to successfully reproduce HIV Gag VLP behaviour in HeLa/CD169 cells. 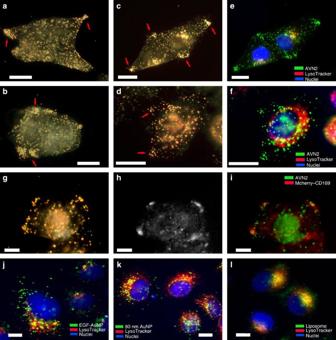Figure 6: GM3-containing AVNs are sequestered in peripheral cellular regions in HeLa/CD169 cells. (a–d) Darkfield images of HeLa/CD169 cells 20 h after an initial 10 min exposure to GM3-containing (a,b) AVN1 or (c,d) AVN2. (e,f) Corresponding fluorescence images of HeLa/CD169 with GM3-containing AVN2 after nucleus (blue) and LysoTracker (red) staining. The AVNs show an enrichment in regions that do not co-stain with the LysoTracker. (g) Darkfield, (h) CD169–mCherry fluorescent image and (i) overlay of GM3–AVN2 on HeLa/CD169–mCherry cells 20 h after incubation, which confirms increased CD169 concentrations at locations of AVN2 enrichment. The images in (a–i) show representative cells from five independent experiments. (j–l) Overlaid darkfield (green) and fluorescence LysoTracker images (red) of HeLa/CD169 cells after (j) 4 h of incubation with epidermal growth factor functionalized 80 nm Au NPs, (k) 20 h after incubation with pegylated 80 nm Au NPs, or (l) 20 h after 10 min incubation with fluorescently labelled GM3–liposomes. Scale bars, 10 μm. Figure 6: GM3-containing AVNs are sequestered in peripheral cellular regions in HeLa/CD169 cells. ( a – d ) Darkfield images of HeLa/CD169 cells 20 h after an initial 10 min exposure to GM3-containing ( a , b ) AVN1 or ( c , d ) AVN2. ( e , f ) Corresponding fluorescence images of HeLa/CD169 with GM3-containing AVN2 after nucleus (blue) and LysoTracker (red) staining. The AVNs show an enrichment in regions that do not co-stain with the LysoTracker. ( g ) Darkfield, ( h ) CD169–mCherry fluorescent image and ( i ) overlay of GM3–AVN2 on HeLa/CD169–mCherry cells 20 h after incubation, which confirms increased CD169 concentrations at locations of AVN2 enrichment. The images in ( a – i ) show representative cells from five independent experiments. ( j – l ) Overlaid darkfield (green) and fluorescence LysoTracker images (red) of HeLa/CD169 cells after ( j ) 4 h of incubation with epidermal growth factor functionalized 80 nm Au NPs, ( k ) 20 h after incubation with pegylated 80 nm Au NPs, or ( l ) 20 h after 10 min incubation with fluorescently labelled GM3–liposomes. Scale bars, 10 μm. Full size image We correlated AVN clustering with the spatial CD169 distribution through combination of darkfield and fluorescence microscopy in HeLa cells expressing CD169–mCherry fusion protein. Analogous to the colocalization of CD169 with HIV Gag–eGFP VLPs ( Fig. 4e–g ), the overlay of darkfield and fluorescence images in Fig. 6g–i reveals an enrichment of CD169 at the sites of AVN clustering. The co-clustering of AVNs and CD169 20 h after AVN binding implies that GM3 remains associated with the NPs after binding to the cell. The demonstration of CD169-dependent binding and spatial clustering of AVNs confirms a successful reproduction of the HIV Gag VLP behaviour in HeLa/CD169. Since GM3 is the only ligand on the AVN surface, and because the non-specific binding of AVNs without GM3 is negligible, the successful reverse engineering of HIV Gag VLPs with AVNs provides direct experimental evidence that GM3−CD169 binding interactions are responsible for triggering the cellular response that culminates in the observed spatial sequestration of HIV Gag VLPs and AVNs. We also emphasize that the spatial redistribution observed for GM3-functionalized AVNs cannot be attributed to a general cellular response to non-degradable inorganic nanomaterials. The spatial sequestration of AVNs is strikingly different from what is typically observed for NPs that undergo conventional endocytosis [60] . Epidermal growth factor functionalized NPs ( Fig. 6j ), which target the endocytic epidermal growth factor receptor, as well as pegylated NPs ( Fig. 6k ), are collected in perinuclear, acidified compartments. Due to the long time gap of 20 h between AVN exposure and analysis of AVN distribution in Fig. 6a–i , we can also exclude the possibility that intermediate endocytosis states are observed for the GM3-containing AVNs. Instead, the unique spatial distribution of the AVNs corroborates the hypothesis that GM3–CD169 binding elicits a distinct cellular response different from conventional endocytosis. Interestingly, this behaviour was found to be specific to AVNs, while GM3-containing liposomes of identical composition were exclusively collected in lysosomal compartments ( Fig. 6l ). This difference between the soft liposomes and the stiffer, metal core containing AVNs indicates a role of the mechanical properties in determining the intracellular fate of virus particles. Although HeLa/CD169 cells are a useful model system to test and calibrate AVNs, it is unclear to what degree the observed spatial segregation of AVNs in HeLa/CD169 cells is relevant in DCs that mediate HIV-1 transinfection. To clarify this question, primary monocyte-derived DCs were matured with Escherichia coli lipopolysaccharides and then incubated with AVNs. While binding of Gal-Cer or blank AVNs to mature DCs was very low (see Supplementary Fig. 6 ), GM3-containing AVNs bound efficiently to mature DCs. 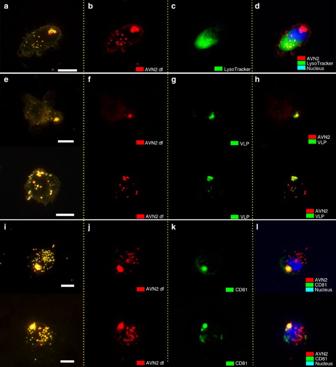Figure 7: Sequestration of GM3-containing AVN2 particles in mature DCs. (a) The colour darkfield image of a representative DC after 1 h of incubation shows a distinct AVN cluster in a peripheral position. The overlay of (b) monochromatic darkfield and (c) LysoTracker images in (d) shows that AVNs are not sequestered into lysosomes. (e) Colour darkfield, (f) monochromatic darkfield and (g) fluorescence images of DCs co-incubated with Gag–eGFP VLPs for 1 h. (h) The overlay of darkfield and fluorescence images confirms that areas enriched in AVNs and VLPs colocalize. (i) Colour darkfield, (j) monochromatic darkfield and (k) fluorescence images of DCs incubated with AVNs and then fluorescently labelled for CD81. (l) The overlay images reveal that AVN-containing compartments are associated with CD81. Scale bars, 5 μm. All DC experiments were independently repeated with primary cells from at least two donors. Figure 7 shows darkfield and fluorescence images of mature DCs that were continuously incubated with GM3-containing AVN1 for 1 h under culture conditions similar to those for HeLa/CD169 cells. We observed that GM3–AVNs captured by mature DCs were redistributed and collected in tightly focused spatial locations. For mature DCs, 1 h of incubation with AVNs was sufficient to result in a strongly polarized AVN distribution with large NP clusters preferentially located at the cell periphery ( Fig. 7a ). Darkfield and fluorescent LysoTracker co-staining experiments ( Fig. 7b–d ) confirm that the AVN-enriched compartments in mature DCs are distinct from lysosomal compartments since no colocalization was observed between AVNs and lysosomal marker. While in HeLa/CD169 cells, multiple smaller AVN clusters are frequently found within a single cell, in mature DCs, we preferentially observed the formation of one single compartment highly enriched in AVNs. Although the data obtained with both mature DCs and HeLa/CD169 cells confirm the existence of a cellular process that results in a spatial coalescence of bound AVNs, CD169-mediated trafficking and localization of AVNs in peripheral non-lysosomal compartments occur with faster kinetics and is more pronounced in mature DCs. Figure 7: Sequestration of GM3-containing AVN2 particles in mature DCs. ( a ) The colour darkfield image of a representative DC after 1 h of incubation shows a distinct AVN cluster in a peripheral position. The overlay of ( b ) monochromatic darkfield and ( c ) LysoTracker images in ( d ) shows that AVNs are not sequestered into lysosomes. ( e ) Colour darkfield, ( f ) monochromatic darkfield and ( g ) fluorescence images of DCs co-incubated with Gag–eGFP VLPs for 1 h. ( h ) The overlay of darkfield and fluorescence images confirms that areas enriched in AVNs and VLPs colocalize. ( i ) Colour darkfield, ( j ) monochromatic darkfield and ( k ) fluorescence images of DCs incubated with AVNs and then fluorescently labelled for CD81. ( l ) The overlay images reveal that AVN-containing compartments are associated with CD81. Scale bars, 5 μm. All DC experiments were independently repeated with primary cells from at least two donors. Full size image We correlated the spatial distributions of VLPs and AVNs in mature DCs through combined fluorescence and darkfield microscopy after 1 h of incubation. We found that the regions enriched in VLPs and AVNs show an almost perfect colocalization ( Fig. 7e–h ), confirming that both VLPs and AVNs are sequestered into identical compartments. Previous studies have demonstrated that cellular compartments containing infectious HIV-1 particles in mature DCs are enriched in tetraspanins [61] , [62] . We immunolabelled the tetraspanin CD81 and imaged its distribution through fluorescence microscopy. These experiments revealed an unambiguous association of CD81 with AVN-containing compartments ( Fig. 7i–l ). Localization of AVNs in HeLa/CD169 cells via FIB/SEM The multimodal Au core of AVNs makes it possible to investigate the peripheral accumulation of AVNs observed in the optical microscope via scanning electron microscopy (SEM) and focused ion beam (FIB) milling [63] . SEM detects the secondary electrons generated on impact from a primary electron beam. Since the secondary electrons have a very short escape depth [64] , SEM imaging is highly surface specific. 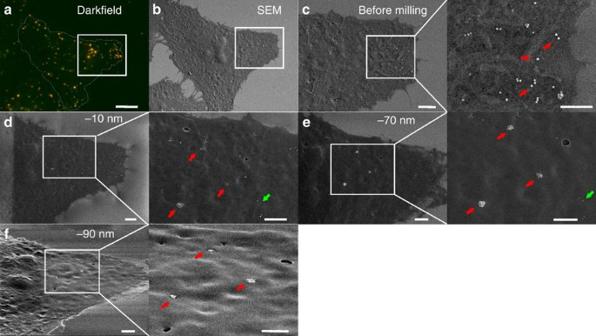Figure 8: SEM/FIB of HeLa/CD169 cells 20 h after exposure to GM3-containing AVN2. (a) Darkfield image of a representative cell with AVN2 clusters. (b) SEM image of the same cell after drying and coating with a 5 nm thin Au/Pd layer. (c) Magnified SEM image of the cell surface in the area of interest marked with a white square in (a,b). The magnified view shows AVN2 particles and clusters located on the cell surface. (d) After removal of ~\n10 nm of cellular material through FIB milling, more clustered (red arrow) and individual (green arrow) AVN2 particles emerge. (e) After an additional removal of ~\n60 nm, the AVN2 clusters (red arrow) and monomers (green arrow) are all completely excavated. (f) SEM image of the area of interest recorded with a tilt angle of 52° after removal of another ~\n20 nm cellular material. No additional AVN2 are exposed. Scale bars, 5 μm for (a,b), and 2 μm for (c,f). Figure 8 shows an optical darkfield ( a ) and correlated SEM ( b ) image of a representative HeLa/CD169 cell 20 h after addition of AVN2. The optical image indicates a large number of bound AVNs and their clustering in a peripheral cell area (white square in Fig. 8a ). A SEM image of the entire cell is shown in Fig. 8b . Before any FIB milling, the number of detected NPs in this area is low, and those NPs that are detected are located right at the cell edge where the cell is very thin ( Fig. 8c ). To obtain further information about the relative localization of the AVN clusters with regard to the cell membrane, we removed cellular material through FIB milling in the area under investigation. Figure 8d and the magnified view show that already after the removal of only 10 nm of cellular material, additional AVN clusters (red arrows) as well as individual AVNs (green arrows) become detectable in areas that did not contain NPs in Fig. 8c . Some clusters are only faintly visible, indicating that they are still mostly contained in the cell matrix. An additional milling of 60 nm further excavates the large AVN clusters ( Fig. 8e ). A tilted view (52°) of the area after removal of ~\n90 nm of cellular material is included in Fig. 8f . When we milled even deeper, the AVNs were gradually removed and no additional AVNs were observed in the investigated cell section. Figure 8: SEM/FIB of HeLa/CD169 cells 20 h after exposure to GM3-containing AVN2. ( a ) Darkfield image of a representative cell with AVN2 clusters. ( b ) SEM image of the same cell after drying and coating with a 5 nm thin Au/Pd layer. ( c ) Magnified SEM image of the cell surface in the area of interest marked with a white square in ( a , b ). The magnified view shows AVN2 particles and clusters located on the cell surface. ( d ) After removal of ~\n10 nm of cellular material through FIB milling, more clustered (red arrow) and individual (green arrow) AVN2 particles emerge. ( e ) After an additional removal of ~\n60 nm, the AVN2 clusters (red arrow) and monomers (green arrow) are all completely excavated. ( f ) SEM image of the area of interest recorded with a tilt angle of 52° after removal of another ~\n20 nm cellular material. No additional AVN2 are exposed. Scale bars, 5 μm for ( a , b ), and 2 μm for ( c , f ). Full size image The picture that emerges from our combined optical and electron microscopic characterization is that, in HeLa/CD169 cells, the GM3–CD169-mediated AVN sequestration at the cell periphery leads to localization of AVN clusters within tens of nanometres below the plasma membrane. At the very edge of the cell, where the cell is thinnest, the AVNs can be located directly on the cell surface. The observation of AVN enrichment close to the membrane in HeLa/CD169 cells warrants additional future studies into the spatial localization of GM3-functionalized AVNs in DCs, where the dynamic range of possible separations between AVNs and plasma membrane is much larger. Our studies also suggest that AVNs in combination with SEM/FIB as an invaluable tool in future studies to determine the localization of GM3-functionalized AVNs in DCs. Self-assembled biomimetic nanosystems with defined surface properties represent engineerable model systems for characterizing the role of specific surface functionalities in virus–host cell interactions. We have used this approach to validate the role of GM3 in the viral envelope glycoprotein-independent binding and cellular trafficking of HIV-1 via a reverse engineering approach. Our observations that GM3 loaded AVNs are sequestered into the same compartments as VLPs and that these compartments are associated with tetraspanins provide experimental evidence for an imitation of virus particle behaviour by AVNs [61] , [62] . The successful mimicry of HIV-1 trafficking mechanisms in monocyte-derived DCs and HeLa/CD169 cells with AVNs that contain only GM3 as a potential ligand unambiguously confirms the hypothesis that GM3 is the non-virus-encoded surface functionality that facilitates an envelope protein-independent capture of HIV-1 particles. Since the AVNs generated in this work share similarities with GM3-presenting exosomes [7] , [9] , our findings are consistent with the Trojan exosome hypothesis [65] that HIV has parasitized host intercellular vesicle trafficking pathways to enhance its dissemination. We implemented two types of GM3-containing AVNs, one containing a complete lipid bilayer membrane (AVN1) and the other containing a single-lipid layer grafted onto the NP surface through hydrophobic interactions (AVN2). The fact that both GM3-functionalized AVN1 and AVN2 bind to HeLa/CD169 but not HeLa cells confirms that CD169 is the receptor for nanoconjugated GM3, independent of its presentation in a lipid monolayer or bilayer. Both types of AVNs were found to elicit a unique spatial sequestration in both HeLa/CD169 and mature DCs. Based on the particle distribution obtained by darkfield imaging, AVN clustering occurs preferentially in peripheral cell areas for both mature DCs and HeLa/CD169 cells. Combined SEM/FIB investigations in HeLa/CD169 cells substantiated this finding by revealing an accumulation of AVN clusters within tens of nanometres below the plasma membrane. In principle, this enrichment of the AVNs in direct vicinity of the plasma membrane could be the result of an exocytic intracellular pathway that directs a significant fraction of endocytosed AVNs from multivesicular endosomes to the plasma membrane via exosomes, especially in immature DCs [7] , [66] . Recent studies have, however, questioned, the role of the exocytic mechanisms in the peripheral sequestration of HIV in mature DCs [67] and, instead, suggested capture and retention of virus in solvent accessible plasma membrane invaginations [62] , [68] . While the localization of virus particles in solvent accessible membrane invaginations is considered essential for efficient inter-cell transfer of viral particles during transinfection [62] , the mechanism by which CD169 traffics virus particles to these peripheral compartments remains unclear. Independent of the exact mechanisms underlying the collection of AVNs in peripheral clusters, the fact that the GM3 containing minimalistic AVNs induce this unique spatial distribution in HeLa/CD169 cells provides experimental evidence in support of the hypothesis that GM3–CD169 interactions play a key role in orchestrating the cellular response of DCs during HIV-1 transinfection [8] , [9] , [12] , [13] , [69] . Interestingly, GM3–CD169 binding can induce this cellular programme despite the absence of any previously defined endocytotic motifs in the cytoplasmic tail of CD169 (ref. 70 ). The dynamics of the spatial sequestration of AVNs and VLPs in HeLa/CD169 cells was found to be slower and the extent less significant than in mature DCs. VLP/AVN clustering in peripheral compartments in HeLa/CD169 cells was apparent at 20 h post VLP/AVN exposure ( Figs 4c,d and 6a–i ). The lack of endocytotic motifs in the cytoplasmic tail of CD169, together with the observation that the sequestration kinetics of AVNs are significantly faster in mature DCs (within 1 h; Fig. 7 ) than in HeLa/CD169, points towards the existence of yet to be identified membrane associated co-factors or mechanisms that accelerate virus uptake and processing after GM3–CD169 engagement in mature DCs. The fact that in HeLa/CD169 a sequestration was observed for GM3-containing AVNs but not for GM3-functionalized liposomes indicates that the presentation of GM3 is necessary but not sufficient to trigger sequestration. One striking difference between AVNs and liposomes of identical size and membrane composition is the difference in structural stiffness. Liposomes [57] are much softer than HIV virions [39] or metal NP [56] containing AVNs. One conclusive rationalization of the differences between liposomes and AVNs is, therefore, that mechanical properties also influence the intracellular fate of virus particles and that—unlike the AVNs—the liposomes are too soft to induce the sequestration observed for the virus. The observed differences in the spatiotemporal distribution of AVNs and liposomes argue in favour of AVNs as the more realistic model system for validating the potential role of specific membrane functionalities in the HIV-1 transinfection mechanism. In addition, AVNs have the advantage that they are multimodal and can be imaged with high contrast in both optical and electron microscopy. The experimental validation that GM3-functionalized AVNs successfully mimic viral behaviour has important implications beyond elucidating fundamental mechanistic details of the GM3–CD169-mediated transfection pathway. A selective capture of GM3–AVNs by CD169 paves the path to new delivery strategies that can selectively deliver drugs and vaccines to CD169-expressing DCs and macrophages in vivo , which are key components of the immune system. Furthermore, our experimental findings show vividly that in contrast to endocytosis and targeting to lysosomal compartments, alternative cellular uptake and trafficking mechanisms can be targeted by smart NPs with rationally designed lipid membrane surfaces. The successful mimicry of HIV-1 sequestration into peripheral non-lysosomal compartments, an evolutionary optimized viral strategy for avoiding lysosomal degradation, forms the basis for novel AVN-based delivery strategies that can minimize the intracellular degradation of sensitive cargo. Due to their ability to target key cells of the immune system and to initiate non-lysosomal uptake routes, GM3-functionalized AVNs can contribute significantly to overcome key challenges in drug delivery. AVN1 preparation (strategy S1) A volume of 1 ml 1.1 × 10 10 particles ml −1 colloidal Au NPs with a nominal diameter of 80 nm (Ted Pella) were incubated with 5 μl of 10 mM polyethylene glycol thiol propionic acid (acid–PEG) overnight, followed by three cycles of washing through centrifugation (600 g , 10 min) and resuspension in double distilled (ddi) water to remove excess acid–PEG. The functionalized Au NPs were resuspended into 1 ml of 10 mM NaCl, pH=7. Simultaneously, a total amount of 1 μmol of lipid mixture (Avanti Polar Lipids, Alabaster, AL) (major components are dipalmitoylphosphatidylcholine, cholesterol and phosphatidylserine, GM3 or Gal-Cer; details in Table 1 ) was dissolved in 100 μl chloroform in a clean 25 ml round-bottom flask. The flask containing the lipid mixture was then sonicated briefly for 5 s with a bath sonicator (Branson 5510), followed by rotary evaporation for 15 min. A uniformly thin lipid dry layer formed on the bottom of the flask, which was further dried under vacuum overnight. The above acid–PEG-functionalized Au NPs solution was injected into the flask through a disposable syringe to rehydrate the lipid film in the presence of Au NPs at 50 °C for 1 h. Subsequently, 30-min sonication was applied to agitate the suspension and maximize lipid hydration. Immediately after sonication, the lipid–Au NP mixture was transferred into a cryo-vial under Ar protection, and underwent three freeze–thaw cycles in liquid nitrogen and 50 °C water. After another sonication step of 30 min, the solution was extruded through a 200 nm pore size polystyrene membrane with a mini extruder set (Avanti Polar Lipids). AVNs were then purified from free liposomes through three cycles of centrifugation (600 g , 10 min), and resuspended in 100 μl per 10 mM NaCl for further use. AVN2 preparation (strategy S2) A thin dry layer of lipid mixture was prepared following the procedures described for AVN1. A volume of 1 ml of 20 mM HEPES buffer (pH=7.2) was then added, forming a cloudy solution after vigorous agitation. The mixture was then sonicated for 30 min in ice bath until the solution became clear. This liposome solution was then stored in 4 °C for further use. A volume of 1 ml of 100 nm colloidal Au NP solution (1.1 × 10 10 particles ml −1 ) was pelleted via centrifugation at 600 g for 10 min. A volume of 0.5 ml of the prepared liposome solution was added to the Au pellet, and the volume was increased to 1 ml with 20 mM HEPES buffer. A volume of 200 μl of 0.01 mg ml −1 1-octadecanethiol solution in ethanol was then added dropwise to the mixture. The mixed solution was agitated overnight on a rotator. After that, the AVNs were washed three times through centrifugation (600 g , 10 min) and resuspended in ddi water. Finally, the AVN pellet was resuspended in 100 μl 20 mM HEPES buffer and ready to use. TEM characterization of AVNs AVN stock solutions were diluted to ~\n1 × 10 7 AVNs ml −1 with ddi water and drop-cast onto carbon-coated TEM grids. Excess solution was removed by a clean filter paper after 1-min incubation, and the samples were dried and stored in vacuum before imaging using a JEOL JEM 2010 HRTEM with 200 kV HT. Ultraviolet–vis Spectra of diluted AVN solutions (1 × 10 7 particles ml −1 ) in 10 mM NaCl (pH=7.0) were acquired on an Agilent Cary 5000 UV/VIS spectrometer. 10 mM NaCl was used for baseline correction. All spectra were normalized relative to their peak maxima. Dynamic light scattering and zeta potential measurements Measurements were performed on a Zetasizer Nano ZS90 (Malvern, Worcestershire, UK). AVNs were diluted to 1 × 10 7 particles ml −1 with 10 mM NaCl (pH=7.0). Cells and cell culturing HeLa/CD169 cells stably expressing CD169 were established by transduction with VSV–G pseudotyped LNC–CD169 retroviral vector as described in Puryear et al . [13] CD169 expression was confirmed by flow cytometry and immunofluorescence assay with Alexa-647 conjugated anti-CD169 antibody (AbD-Serotec; 1:50 dilution). Note that ~\n60% of cells expressed CD169 (see Supplementary Fig. 5a,b ). To generate CD169–mCherry fusion protein, the ApaI-XbaI fragment containing 3′ half of CD169 from LNC–CD169 was subcloned into the pSL1180 vector (GE Healthcare Life Science), and the stop codon of CD169 mutated to glycine (from TGA to GGA) by PCR using the following primers, CD169-4188-F (5′-ATCAGGGACAGGCCATGTCC-3′) and CD169-stop-R (5′-ACCTCTAGACAACACCACTGGTCCGCCCAGG-3′). The mutagenized fragment was cloned back into the corresponding region of CD169 in LNC-CD169 using SbfI and XbaI restriction sites. To create an XbaI site at the 5′ end of the mCherry gene, the mCherry gene was amplified from Gag–mCherry-encoding plasmid [7] by PCR using the following primers, GFP-5-XbaI-F (5′-AAAAAATCTAGAATGGTGAGCAAGGG-3′) and Gag–eGFP-N-R (5′-AACCTCTACAAATGTGGTATGG-3′). The PCR-amplified mCherry gene was digested with XbaI and NotI, and cloned in frame into the carboxy-terminal end of the stop-codon-mutated-CD169 (LNC–CD169–mCherry). HeLa cells were transduced with LNC–CD169–mCherry retroviral vector as described previously [13] , selected and maintained in the presence of 0.5 mg ml −1 G418 (Life Technologies). Both HeLa/CD169 cells and HeLa/CD169–mCherry cells were cultured in 10% fetal bovine serum, 1% penicillin–streptomycin and 0.5 mg ml −1 G418-containing DMEM. Primary monocyte-derived DCs were differentiated from CD14 + peripheral blood monocytes and matured with lipopolysaccharides (100 ng ml −1 ) for 2 days as described elsewhere [7] , [13] . Both HeLa/CD169 cells and HeLa/CD169–mCherry cells were cultured in 10% fetal bovine serum, 1% penicillin–streptomycin and 0.5% G418-containing DMEM. VLP generation HIV Gag–eGFP VLPs were obtained by transient (calcium phosphate-mediated) transfection of HEK293T cells with the pGag–eGFP plasmid expressing codon-optimized Gag–eGFP fusion protein [13] . VLP-containing cell-free supernatants were collected 2 days post transfection, cleared of cell debris by filtration through 0.45 μm filters, aliquoted and stored at −80°C until use. AVN and VLP binding and sequestration Before exposure to AVNs or VLPs, HeLa/CD169 cells were seeded on 24 × 60 mm 2 coverslips and cultured to 30–40% confluency. The cell coverslips were then briefly rinsed with warm Hank’s buffer (no Ca 2+ /Mg 2+ ) (Life Technologies). AVNs or VLPs were diluted to 5 × 10 8 particles ml −1 (AVN) or 1 × 10 10 particles ml −1 (VLPs) with DMEM, and 1 ml of diluted AVNs or VLPs was added to the coverslips and incubated at 37 °C for the specified time in a water-saturated atmosphere with 5% CO 2 . Excess AVNs or VLPs were subsequently removed by washing with warm Hank’s buffer for three times. For binding studies, the cells were then fixed with 4% paraformaldehyde and imaged. In experiments monitoring the temporospatial redistribution of the AVNs or VLPs, excess particles were removed after 10-min incubation and the cells were reimmersed into complete growth medium and further incubated at 37 °C. After 20 h, the cells were treated with 100 nM LysoTracker Deep Red (Invitrogen) and nucleus stain Hoechst 33,342 for 30 min at 37 °C. Samples were then washed with Hank’s buffer and fixed by 4% paraformaldehyde for 15 min at room temperature and subsequently imaged. For DC samples, AVNs were incubated with DCs for 1 h at 37 °C, and washed with 1 × PBS buffer by centrifugation for three times. Cells were then fixed by 4% paraformaldehyde and cytospun onto poly- L -lysine-treated glass coverslips (Sigma). For colocalization of GM3–AVNs and HIV Gag–eGFP VLPs in mDCs, cells were challenged with 10 7 AVN2 particles and 5 × 10 9 VLPs for 1 h at 37 °C, washed, fixed with 4% paraformaldehyde and processed for imaging as described above. To determine if GM3–AVN2 were co-localized with CD81 in mDCs, cells were challenged with 10 7 AVN2 for 1 h at 37 °C, fixed with 4% PFA, permeabilized with 0.5% Triton X-100, blocked with 20% normal human serum and stained with α-CD81 mAb (BD; 1:50 dilution) and detected with Alexa488-conjugated secondary antibody (Invitrogen; 1:50 dilution), as described previously [13] . For SEM/FIB microscopy, cell samples were fixed with 2.5% glutaraldehyde solution for 15 min at room temperature and dehydrated by gradient concentrations of acetone (30%, 50%, 70%, 95%, 100%, 15 min each) and subsequent vacuum drying. Samples were stored in desiccators and sputter coated with 5 nm Au/Pd before SEM/FIB. Image recording and data processing All optical imaging experiments were performed on an Olympus IX71 inverted microscope (see Supplementary Fig. 3 ). Images were taken with a 60 × oil objective with variable NA (NA=0.65–1.25). For darkfield imaging, the samples were illuminated with a 100 W tungsten lamp through a high NA oil darkfield condenser (NA=1.2–1.4). Darkfield images were recorded with an Olympus SP310 digital camera or Nikon D3100 SLR connected to the microscope through an eyepiece adaptor. Fluorescence imaging was performed under epi-illumination using appropriate filter sets. Images were recorded with an Andor Ixon + electron multiplying charge coupled device detector. The NA of the collecting objective was adjusted for darkfield and fluorescence imaging to optimize signal to noise. The recorded images were further processed by ImageJ for coordinate alignment and overlay. SEM/FIB and correlation with optical microscopy Cell dishes intended for characterization through SEM/FIB were diced into 1 cm × 1 cm squares, and covered by a SEM finder grid (SEMF2, copper, Ted Pella). The grid was immobilized through super glue. Ethanol was dropped onto the sample to locate cells of interest in darkfield microscopy. The samples were then dried, and sputter coated with a ~\n5 nm thick Au/Pd layer to increase conductivity. Samples were kept in desiccators until they were transferred into the SEM/FIB. To mount the sample, conductive copper tape was used to attach the coated sample onto SEM stub, and carbon paint was used to increase the conductivity. Samples were imaged first using a Zeiss Supra40VP SEM at 2.0 kV and a working distance of 6 mm. The samples were subsequently milled and imaged with an FEI Quanta 3D FIB instrument. The milling was done with 30 kV 0.5nA Gallium ion beam with 20-s intervals. The estimated milling depth per step was calibrated by applying the same milling on a spin-coated PMMA chip and measuring the resulting depth with a Zygo Optical Profiler (New View 6300). How to cite this article : Yu, X. et al . Glycosphingolipid-functionalized nanoparticles recapitulate CD169-dependent HIV-1 uptake and trafficking in dendritic cells. Nat. Commun. 5:4136 doi: 10.1038/ncomms5136 (2014).